A non-canonical function of telomerase RNA in the regulation of developmental myelopoiesis in zebrafish Dyskeratosis congenita (DC) is an inherited disorder with mutations affecting telomerase or telomeric proteins. DC patients usually die of bone marrow failure. Here we show that genetic depletion of the telomerase RNA component ( TR ) in the zebrafish results in impaired myelopoiesis, despite normal development of haematopoietic stem cells (HSCs). The neutropenia caused by TR depletion is independent of telomere length and telomerase activity. Genetic analysis shows that TR modulates the myeloid–erythroid fate decision by controlling the levels of the master myeloid and erythroid transcription factors spi1 and gata1 , respectively. The alteration in spi1 and gata1 levels occurs through stimulation of gcsf and mcsf . Our model of TR deficiency in the zebrafish illuminates the non-canonical roles of TR , and could establish therapeutic targets for DC. Telomerase is a RNA-dependent DNA polymerase that synthesizes telomeric repeats at the end of eukaryotic chromosomes [1] . This enzyme complex consists of a catalytic protein with a telomere-specific reverse transcriptase activity (TERT), an internal RNA template (TR) and a number of associated proteins [2] . Telomerase is essential for the lifelong maintenance of multiple cells, including haematopoietic stem cells (HSCs) [3] . Traditionally, telomerase alterations have been associated to cancer and aging. TERT, TR or both components are also involved in some rare human diseases. For example, heterozygous mutations of human TR and TERT genes have been described in patients with acquired aplastic anaemia and the autosomal dominant form of dyskeratosis congenita (DC) [4] , [5] and in patients with idiopathic pulmonary fibrosis [6] . DC is an inherited disorder characterized by a variety of phenotypes but patients usually die of bone marrow failure [7] . DC patients show signs of premature aging and they are more susceptible to develop cancers. All DC patients have some defects in telomere biology and those defects affect the renewing capabilities of HSCs [8] , [9] . All mutations identified to date in DC patients are found in telomerase components or in telomere-stabilizing components [7] . Although mutations in both TR and TERT genes act as autosomal dominant due to an haploinsufficiency of telomerase and show disease anticipation associated with progressive telomere shortening [10] , the presentation of the disease is more serious in patients with mutations affecting TR [7] . Besides its telomere-lengthening function, there is increasing evidence that TERT can have physiological roles that are independent of this central function in both mammals [11] , [12] , [13] , [14] , [15] and zebrafish [16] . Zebrafish telomerase promotes the development of haematopoietic cells through a non-canonical mechanism that is independent of the authentic telomerase activity of TERT and the role of this enzyme in telomere lengthening [16] . The cancer-promoting activity of TR may occur independently of telomerase activity [17] , [18] , [19] , [20] . Although the mechanism involved in this activity of TR is largely unknown, a recent study identified 2,198 TR-binding sites in the genome using chromatin isolation by RNA purification (ChIRP), which represents a large resource to study potential non-canonical functions of TR RNA and telomerase [21] . TR occupied multiple Wnt genes directly and several binding sites near the MYC gene, concordant with previously documented binding sites of TERT [21] . In the present study, we have taken advantage of the easy genetic manipulation and transparency of zebrafish embryos, together with the availability of several transgenic lines with labelled blood cells, to identify a non-canonical role of TR. Genetic inhibition of TR demonstrated normal emergence of HSCs, but there is an alteration of cell fate. The change in developmental myelopoiesis occurs through the regulation of the master myeloid and erythroid transcription factors spi1 and gata1. The alteration in levels of these transcription factors is controlled by the stimulation of granulocyte- and macrophage colony-stimulating factors. Telomere length in the TR -deficient animals is surprisingly normal. Our studies identify a cell fate change established by a non-canonical role for TR . TR deficiency impairs telomerase activity To study the role of telomerase RNA component ( TR ) in haematopoiesis, we used antisense morpholino (MO)-mediated knockdown technology in zebrafish embryos. Three different MOs were designed, each one targeting a different domain of TR , namely the template, CR4/CR5 and ScaRNA domains ( Fig. 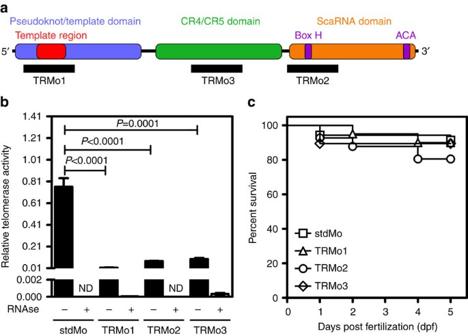Figure 1:TRdeficiency impairs telomerase activity. (a) Scheme showing the location of the different MOs against zebrafishTR. The different domains are according to Xieet al.63(b) Zebrafish embryos were microinjected at the one-cell stage with stdMo or the three different MOs againstTR. At 3 dpf, telomerase activity was measured by Q-TRAP in 100 pooled zebrafish larvae using 1 μg of protein extract. The specificity of the assay was confirmed using negative control samples that were treated with 1 μg of RNAse at 37 °C for 20 min. Results are expressed as the mean±s.e.m. from triplicate samples. Statistical significance was assessed using the Student’st-test (P<0.05). ND: not detected. (c) Kaplan–Meier representation of the survival of three genetic backgrounds (stdMo,n=35; TRMo1,n=20; TRMo2,n=41; TRMo3,n=38). The survival curves were not statistically different, log rank testP>0.05. 1a , Supplementary Table 1 ). The efficiency of these MOs was assayed by quantitative telomeric repeat amplification protocol (Q-TRAP) ( Fig. 1b ), which has been reported to be a rapid and accurate assay for the quantification of telomerase activity [22] . In each case, there was impaired telomerase activity, yet none of the MOs significantly affected zebrafish survival for up to 5 days ( Fig. 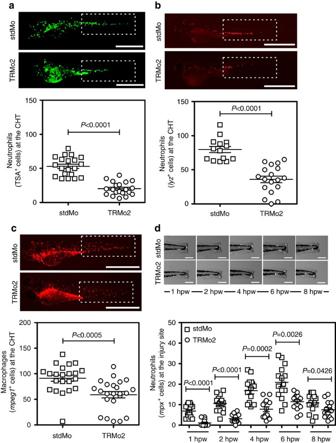Figure 2:TRdeficiency induces neutropenia and monocytopenia but does not compromise neutrophil functionality. Zebrafish embryos were microinjected at the one-cell stage with stdMo or TRMo2. At 3 dpf, neutrophils were stained using the TSA kit (a) or directly visualized in Tg(lyz::DsRed) fish (b) by fluorescence microscopy and manually counted at the CHT. (c) Macrophages of 3 dpf Tg(mpeg1::mCherry) were similarly visualized under fluorescence microscopy and counted at the CHT. (d) Tailfins of Tg(mpx::eGFP) std andTRmorphants were transected at 3 dpf and the number of fluorescent neutrophils visible in the tail was assessed by fluorescence microscopy. Positive cells in animals from both groups were visually quantified from high-quality pictures from an 8 h time series. Each symbol represents one larva and the mean±s.e.m. is also indicated. (a) stdMo,n=20; TRMo2,n=20. (b) stdMo,n=14; TRMo2,n=15. (c) stdMo,n=22; TRMo2,n=23. (d) stdMo,n=15; TRMo2,n=14. Statistical significance was assessed using the Student’st-test (P<0.05). Scale bars, 1 mm (a–c) and 0.2 mm (d). hpw, hours post wounding. 1c ) nor altered development ( Supplementary Table 2 ). Figure 1: TR deficiency impairs telomerase activity. ( a ) Scheme showing the location of the different MOs against zebrafish TR . The different domains are according to Xie et al. [63] ( b ) Zebrafish embryos were microinjected at the one-cell stage with stdMo or the three different MOs against TR . At 3 dpf, telomerase activity was measured by Q-TRAP in 100 pooled zebrafish larvae using 1 μg of protein extract. The specificity of the assay was confirmed using negative control samples that were treated with 1 μg of RNAse at 37 °C for 20 min. Results are expressed as the mean±s.e.m. from triplicate samples. Statistical significance was assessed using the Student’s t -test ( P <0.05). ND: not detected. ( c ) Kaplan–Meier representation of the survival of three genetic backgrounds (stdMo, n =35; TRMo1, n =20; TRMo2, n =41; TRMo3, n =38). The survival curves were not statistically different, log rank test P >0.05. Full size image TR deficiency induces neutropenia Although TR knockdown with three different MOs had no obvious effect on development, blood cell formation and circulation, we analysed in more detail the number of neutrophils at the caudal haematopoietic tissue (CHT) at 3 days post fertilization (dpf) using a Tyramide Signal Amplification (TSA) staining assay for the detection of myeloperoxidase (Mpx) [23] , which is a specific marker of zebrafish neutrophils [24] . Interestingly, the three TR morphants showed a marked neutropenia compared with the control group ( Fig. 2a and Supplementary Fig. 1 ). To rule out that TR deficiency directly affected the expression or activity of Mpx, rather than neutrophil development and maintenance, we directly counted the number of lysozyme positive cells in the tg( lyz :DsRed) line, which has red fluorescent neutrophils [25] , and neutropenia was evident ( Fig. 2b ). To examine whether macrophages were affected, a tg( mpeg1 :mCherry) line was used that has red fluorescent macrophages [26] . The number of macrophages was also reduced in TR -deficient larvae ( Fig. 2c ). Figure 2: TR deficiency induces neutropenia and monocytopenia but does not compromise neutrophil functionality. Zebrafish embryos were microinjected at the one-cell stage with stdMo or TRMo2. At 3 dpf, neutrophils were stained using the TSA kit ( a ) or directly visualized in Tg( lyz ::DsRed) fish ( b ) by fluorescence microscopy and manually counted at the CHT. ( c ) Macrophages of 3 dpf Tg( mpeg1 ::mCherry) were similarly visualized under fluorescence microscopy and counted at the CHT. ( d ) Tailfins of Tg( mpx ::eGFP) std and TR morphants were transected at 3 dpf and the number of fluorescent neutrophils visible in the tail was assessed by fluorescence microscopy. Positive cells in animals from both groups were visually quantified from high-quality pictures from an 8 h time series. Each symbol represents one larva and the mean±s.e.m. is also indicated. ( a ) stdMo, n =20; TRMo2, n =20. ( b ) stdMo, n =14; TRMo2, n =15. ( c ) stdMo, n =22; TRMo2, n =23. ( d ) stdMo, n =15; TRMo2, n =14. Statistical significance was assessed using the Student’s t -test ( P <0.05). Scale bars, 1 mm ( a – c ) and 0.2 mm ( d ). hpw, hours post wounding. Full size image We next examined myeloid cell activity in TR -deficient larvae. First, we performed a recruitment assay to study neutrophil responses to an injury by tail fin transaction of 3 dpf mpx ::eGFP zebrafish larvae. Although the neutrophil number at the injury site was lower at all time points analysed in TR -deficient larvae, the kinetics of the recruitment was similar in both groups, being maximum at 6 h post injury ( Fig. 2d ), as previously described [24] . We next infected the larvae with the intracellular pathogenic bacterium S. typhimurium and found that the TR -deficient embryos showed similar resistance to infection with this bacterium ( Supplementary Fig. 2a ). Depletion of myeloid cells, that is, neutrophils and macrophages, using a MO against the master myeloid transcription factor spi1 (also known as pu.1 ) [27] rendered larvae hypersusceptible to S. typhimurium infection ( Supplementary Fig. 2a ). In addition, TR -deficient larvae were also able to respond to S. typhimurium infection by upregulating the expression of the genes encoding the powerful pro-inflammatory cytokines IL-1β and TNFα, albeit at lower levels than their wild-type siblings ( Supplementary Fig. 2b ). Altogether, these observations establish that TR -deficient larvae have reduced number of neutrophils and macrophages, but that the cells that are present are fully functional. TR regulates myelopoiesis independently of telomere length As the knockdown of TR by MOs resulted in the lack of telomerase activity, we wondered whether the use of TR deficiency resulted in the shortening of telomere length, which may explain the observed phenotype. Telomere length was measured by quantitative-fluorescence in situ hybridization (Q-FISH) in interphasic blood cells collected from 3 dpf larvae injected with stdMo and TRMo2. The results showed a similar telomere shortening, weak but significant, in TR - and TERT -deficient larvae ( Fig. 3a and Supplementary Fig. 3a ). In addition, the proportion of blood cells with short telomeres was similar in both groups of animals ( Fig. 3a ). Next, we wondered whether the neutropenia of TR -deficient larvae was related to the lack of telomerase activity. To accomplish this, we performed a TSA staining assay at 30 hpf using a tert −/− zebrafish line, which lack telomerase activity [28] , and their tert +/+ siblings. Although tert -deficient embryos showed normal number of neutrophils, the deficiency of TR resulted in the reduction of neutrophils in both wild type and tert -deficient fish to a similar level, demonstrating that the loss of neutrophils was independent of telomerase activity ( Fig. 3b ). 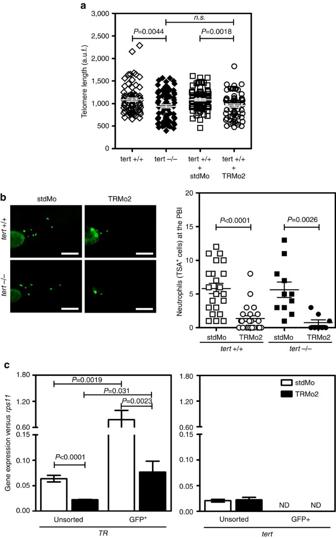Figure 3: The induction of neutropenia byTRdepletion is independent of both telomere length and telomerase activity. Zebrafish embryos were microinjected at the one-cell stage with stdMo or TRMo2. (a) Telomere length was evaluated by Q-FISH in interphasic blood cells from 3 dpf larvae. Each symbol represents one cell and the mean±s.e.m. is also indicated. tert +/+,n=80; tert −/−,n=83; stdMo,n=85; TRMo2,n=68. Statistical significance was assessed using the Student’st-test (P<0.05). (b) Neutrophils oftert+/+ andtert−/− embryos were stained at 30 hpf using the TSA kit, visualized by fluorescence microscopy and manually counted at the PBI. Each symbol represents one embryo and the mean±s.e.m. is also indicated. tert +/+, std Mo,n=22; tert +/+, TRMo2,n=22; tert −/−, stdMo,n=11; tert −/−, TRMo2,n=8. Statistical significance was assessed using the Student’st-test (P<0.05). (c) The mRNA levels ofTRandtertwas determined by RT-qPCR in unsorted versus neutrophils (mpx+) at 3 dpf. The graph shows the mean±s.e.m. of triplicate samples and is representative of three independent experiments. Statistical significance was assessed using the Student’st-test (P<0.05). n.s., not significant; ND, not detected. Scale bars, 200 μm. Figure 3: The induction of neutropenia by TR depletion is independent of both telomere length and telomerase activity. Zebrafish embryos were microinjected at the one-cell stage with stdMo or TRMo2. ( a ) Telomere length was evaluated by Q-FISH in interphasic blood cells from 3 dpf larvae. Each symbol represents one cell and the mean±s.e.m. is also indicated. tert +/+, n =80; tert −/−, n =83; stdMo, n =85; TRMo2, n =68. Statistical significance was assessed using the Student’s t -test ( P <0.05). ( b ) Neutrophils of tert +/+ and tert −/− embryos were stained at 30 hpf using the TSA kit, visualized by fluorescence microscopy and manually counted at the PBI. Each symbol represents one embryo and the mean±s.e.m. is also indicated. tert +/+, std Mo, n =22; tert +/+, TRMo2, n =22; tert −/−, stdMo, n =11; tert −/−, TRMo2, n =8. Statistical significance was assessed using the Student’s t -test ( P <0.05). ( c ) The mRNA levels of TR and tert was determined by RT-qPCR in unsorted versus neutrophils (mpx + ) at 3 dpf. The graph shows the mean±s.e.m. of triplicate samples and is representative of three independent experiments. Statistical significance was assessed using the Student’s t -test ( P <0.05). n.s., not significant; ND, not detected. Scale bars, 200 μm. Full size image The role played by TR in myelopoiesis independently of telomerase activity prompted us to examine the expression of TR and tert genes in sorted neutrophils (mpx + cells) ( Fig. 3c ). TR RNA levels were strikingly higher in neutrophils than in unsorted cells, while tert mRNA was undetectable in neutrophils. Interestingly, the TRMo2 was able to strongly reduce the RNA levels of TR in unsorted cells and neutrophils but had no effect on tert mRNA levels ( Fig. 3c ). As expected, TR ( Supplementary Fig. 3b ) and tert ( Supplementary Fig. 3c ) genes were ubiquitously expressed during development, although tert was found to be expressed at higher levels by skin and neuromasts of 3 dpf larvae. These results further suggest a non-canonical role of TR in myelopoiesis. TR is required for myelopoiesis but dispensable for HSCs To further determine the role of TR in zebrafish definitive haematopoiesis, we analysed the expression of the specific haematopoietic genes lmo2 , gata1a , spi1 ( pu.1 ), gcsfr , cmyb , runx1 and rag1 by using whole-mount in situ hybridization (WISH) at different time points. The expression of lmo2 and gata1a , which are markers of erythromyeloid progenitors (EMPs) at 30 hpf and are expressed in the posterior blood island (PBI) [29] , was unaffected by TR deficiency ( Fig. 4a,b ). The expression of spi1 and gcsfr , canonical markers of myeloid cells and neutrophils, respectively, was severely reduced at the PBI ( Fig. 4c,d ). This result was further confirmed with a TSA staining assay at 30 hpf, which showed the reduction of neutrophils (mpx + cells) in TR -deficient embryos ( Fig. 4e ). The expression of cmyb and runx1 begin by 36 hpf at the aorta–gonad–mesonephros (AGM) and they mark emerging definitive haematopoietic stem and progenitor cells [30] . Notably, the absence of TR did not affect the expression of cmyb and runx1 ( Fig. 4f,g ). This result was also verified using the Tg( cd41 ::eGFP) [31] , in which the number of cd41 + cells (HSCs and thrombocytes) at 3 dpf was independent of the presence of TR ( Fig. 4h and Supplementary Fig. 4a ). Similarly, the expression of gata1a and rag1 , which are expressed in erythrocytes and differentiated thymic T cells, respectively, was apparently unaffected by TR deficiency ( Fig. 4i,j ). Similarly, o-dianisidine staining of the erythroid haemoglobin was also unaltered in TR -deficient embryos ( Supplementary Fig. 4b ). In sharp contrast, the expression of the myeloid markers spi1 ( Fig. 4k,l ) and gcsfr ( Fig. 4m,n ) was significantly reduced at this time. Collectively, these results suggest that although TR is dispensable for the development of EMPs and HSCs in zebrafish embryos, it is required for the differentiation of neutrophils, and likely macrophages, from EMPs and HSCs. 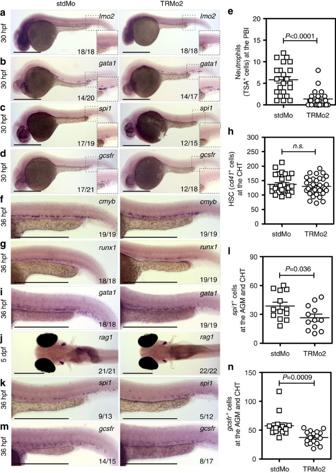Figure 4:TRis required for myelopoiesis but dispensable for the emergence of HSCs. Zebrafish embryos were microinjected at the one-cell stage with stdMo or TRMo2. At the indicated times, whole-mountin situhybridization (WISH) was performed using antisense probes to the indicated haematopoietic genes. Scale bar, 0.5 mm. (a–d) WISH oflmo2,gata1a,spi1andgcsfrgenes at 30 hpf. (e) Neutrophils were stained at 30 hpf and visualized by fluorescence microscope and manually counted at the PBI. (f,g) WISH ofcmybandrunx1genes at 36 hpf. (h) The number ofcd41+ cells of Tg(cd41::eGFP) zebrafish were directly visualized by fluorescence microscopy at 3 dpf and manually counted at the CHT. (i) WISH ofgata1at 36 hpf,rag1at 5 dpf (j) andspi1at 36 hpf (k). (l) Quantification ofspi1+cells at the AGM and CHT at 3 dpf. (m) WISH ofgcsfrat 36 hpf and (n) quantification ofgcsfr+cells at the AGM and CHT at 3 dpf. Numbers in pictures represent the animals with the shown phenotype per total analysed animals. Each symbol in graphs represents one embryo per larva and the mean±s.e.m. is also indicated. (e) stdMo,n=22; TRMo2,n=22. (h) stdMo,n=27; TRMo2,n=34. (l) stdMo,n=13; TRMo2,n=12. (n) stdMo,n=15; TRMo2,n=17. Statistical significance was assessed using the Student’st-test (P<0.05). n.s., not significant. Figure 4: TR is required for myelopoiesis but dispensable for the emergence of HSCs. Zebrafish embryos were microinjected at the one-cell stage with stdMo or TRMo2. At the indicated times, whole-mount in situ hybridization (WISH) was performed using antisense probes to the indicated haematopoietic genes. Scale bar, 0.5 mm. ( a – d ) WISH of lmo2 , gata1a , spi1 and gcsfr genes at 30 hpf. ( e ) Neutrophils were stained at 30 hpf and visualized by fluorescence microscope and manually counted at the PBI. ( f , g ) WISH of cmyb and runx1 genes at 36 hpf. ( h ) The number of cd41 + cells of Tg( cd41 ::eGFP) zebrafish were directly visualized by fluorescence microscopy at 3 dpf and manually counted at the CHT. ( i ) WISH of gata1 at 36 hpf, rag1 at 5 dpf ( j ) and spi1 at 36 hpf ( k ). ( l ) Quantification of spi1 + cells at the AGM and CHT at 3 dpf. ( m ) WISH of gcsfr at 36 hpf and ( n ) quantification of gcsfr + cells at the AGM and CHT at 3 dpf. Numbers in pictures represent the animals with the shown phenotype per total analysed animals. Each symbol in graphs represents one embryo per larva and the mean±s.e.m. is also indicated. ( e ) stdMo, n =22; TRMo2, n =22. ( h ) stdMo, n =27; TRMo2, n =34. ( l ) stdMo, n =13; TRMo2, n =12. ( n ) stdMo, n =15; TRMo2, n =17. Statistical significance was assessed using the Student’s t -test ( P <0.05). n.s., not significant. Full size image To study whether myeloid progenitor differentiation was altered in the absence of TR , we stained blood cells collected by cardiac puncture from 2 dpf embryos with Wright–Giemsa stain and observed alterations in blood cell morphology in TR -deficient embryos ( Supplementary Fig. 5a ). Thus, the blood cells from TR -deficient embryos showed statistically significant lower radius ( Supplementary Fig. 5b ) and higher nucleus/cytoplasm ratio ( Supplementary Fig. 5c ) than their wild-type siblings. These findings are consistent with a delay in differentiation. TR deficiency alters the spi1 / gata1a balance in blood cells spi1 and gata1 are both transcriptional factors essential for the differentiation of HSCs to myeloid and erythroid cells, respectively. The expression of TR , spi1 and gata1a was analysed in the CHT of 2 dpf embryos. The spi1 / gata1a ratio was significantly reduced when TR was depleted ( Fig. 5a and Supplementary Fig. 6 ), usually because spi1 transcript levels decreased and those of gata1a increased ( Fig. 5b ). 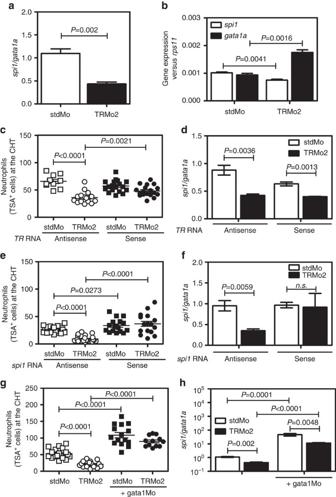Figure 5:TRdeficiency alters the spi1/gata1a balance in blood cells. Zebrafish embryos were microinjected at the one-cell stage with stdMo, TRMo2 or gata1Mo alone or in combination with 50 (spi1) or 200 (TR) pg/egg ofin vitro-transcribed and CAP-modified antisense (as),TRandspi1(sense, s) RNAs. (a)spi1/gata1aexpression ratio (A) and mRNA levels (b) determined by RT-qPCR in tail sections of 2 dpf wild type. The graph shows the mean±s.e.m. of three independent experiments. (c,e,g). Neutrophils were stained at 3 dpf and visualized by fluorescence microscope and manually counted at the CHT. (d,f,h)spi1/gata1aexpression ratio determined by RT-qPCR in tail sections of 2 dpf larvae. Each symbol represents one embryo and the mean±s.e.m. is also indicated. (c) stdMo, RNAas,n=10; TRMo2, RNAas,n=16; stdMo, RNAs,n=18; TRMo2, RNAs,n=18. (e) stdMo, RNAas,n=21; TRMo2, RNAas,n=23; stdMo, RNAs,n=17; TRMo2, RNAs,n=16. Statistical significance was assessed using the Student’st-test (P<0.05). n.s., not significant. Figure 5: TR deficiency alters the spi1/gata1a balance in blood cells. Zebrafish embryos were microinjected at the one-cell stage with stdMo, TRMo2 or gata1Mo alone or in combination with 50 ( spi1 ) or 200 ( TR ) pg/egg of in vitro -transcribed and CAP-modified antisense (as), TR and spi1 (sense, s) RNAs. ( a ) spi1/gata1a expression ratio (A) and mRNA levels ( b ) determined by RT-qPCR in tail sections of 2 dpf wild type. The graph shows the mean±s.e.m. of three independent experiments. ( c , e , g ). Neutrophils were stained at 3 dpf and visualized by fluorescence microscope and manually counted at the CHT. ( d , f , h ) spi1/gata1a expression ratio determined by RT-qPCR in tail sections of 2 dpf larvae. Each symbol represents one embryo and the mean±s.e.m. is also indicated. ( c ) stdMo, RNAas, n =10; TRMo2, RNAas, n =16; stdMo, RNAs, n =18; TRMo2, RNAs, n =18. ( e ) stdMo, RNAas, n =21; TRMo2, RNAas, n =23; stdMo, RNAs, n =17; TRMo2, RNAs, n =16. Statistical significance was assessed using the Student’s t -test ( P <0.05). n.s., not significant. Full size image These results prompted us to investigate the impact of TR overexpression in developmental myelopoiesis. The results showed that an in vitro -transcribed and capped TR RNA was able to rescue the number of neutrophils in TR morphants at 3 dpf ( Fig. 5c ), although it failed to significantly rescue the spi1 / gata1a ratio ( Fig. 5d and Supplementary Fig. 7a ). We next studied the epistatic relationships between TR and spi1 . Overexpression of spi1 RNA was also able to rescue the number of neutrophils ( Fig. 5e ) and the spi1 / gata1a balance ( Fig. 5f and Supplementary Fig. 7b ). Similarly, depletion of gata1a using a specific MO was also able to rescue the number of neutrophils ( Fig. 5g ) and the spi1 / gata1a balance ( Fig. 5h and Supplementary Fig. 7c ). Our studies define a crucial role of TR in maintaining a critical balance between the major myeloid ( spi1 ) and erythroid ( gata1a ) transcription factors. TR regulates the expression of gcsf and mcsf A total of 2,198 TR -binding sites in the human genome have recently been identified, which represent a large resource to study potential non-canonical functions of TR RNA and telomerase [21] . Strikingly, TR occupied binding sites near CSF1 and CSF2 genes, which encode macrophage colony-stimulating factor (MCSF) and granulocyte–macrophage colony-stimulating factor (GMCSF), respectively. Although no orthologues for CSF2 gene have been identified to date in zebrafish, true orthologues for CSF1 and CSF3 , which encode GCSF, have been found and shown to stimulate the survival, proliferation and differentiation of neutrophil and macrophages, respectively [32] , [33] . We sought to determine whether TR was able to regulate the expression of these important cytokines. TR -deficient larvae showed reduced mRNA levels of both gcsf and mcsf compared with wild-type siblings ( Fig. 6a ). Conversely, overexpression of TR RNA increased the transcript levels of both genes ( Fig. 6b ). Overexpression of gcsf ( Fig. 6c ) and mcsf ( Fig. 6d ) mRNAs rescued the number of neutrophils and macrophages, respectively. In addition, gcsf overexpression, and to some extent mcsf , increased spi1 expression levels, while they did not affect TR levels ( Supplementary Fig. 8a,b ). 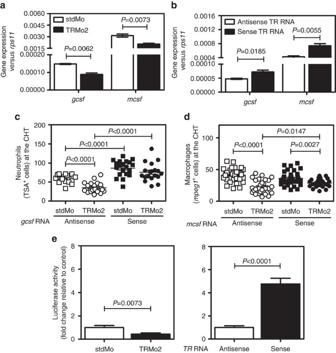Figure 6:TRregulates the expression ofgcsfandmcsf. Zebrafish embryos were microinjected at the one-cell stage with stdMo, TRMo2 (a–e), 100 pg per egg ofin vitro-transcribed and CAP-modified antisense (as),gcsf(c) ormcsf(d) (sense, s) RNAs and/or a 20 pg/egg ofgcsf::Luc and 2 pg/eggRenillaluciferase plasmids (e). (a,b)gcsfandmcsfexpression analysed by RT-qPCR in tail sections of 2 dpf larvae. The graph shows the mean±s.e.m. of three independent experiments. (c,d) Neutrophils were stained at 3 dpf using the TSA kit, visualized by fluorescence microscopy and manually counted at the CHT. Each symbol represents one embryo and the mean±s.e.m. is also indicated. (c) stdMo, RNAas,n=17; TRMo2, RNAas,n=22; stdMo, RNAs,n=20; TRMo2, RNAs,n=19. (d) stdMo, RNAas,n=33; TRMo2, RNAas,n=30; stdMo, RNAs,n=35; TRMo2, RNAs,n=25. (e) Luciferase activity in tail sections of 2 dpf larvae. The graph shows the mean±s.e.m. of three independent experiments performed with triplicates samples. Statistical significance was assessed using the Student’st-test (P<0.05). Figure 6: TR regulates the expression of gcsf and mcsf . Zebrafish embryos were microinjected at the one-cell stage with stdMo, TRMo2 ( a – e ), 100 pg per egg of in vitro -transcribed and CAP-modified antisense (as), gcsf ( c ) or mcsf ( d ) (sense, s) RNAs and/or a 20 pg/egg of gcsf ::Luc and 2 pg/egg Renilla luciferase plasmids ( e ). ( a , b ) gcsf and mcsf expression analysed by RT-qPCR in tail sections of 2 dpf larvae. The graph shows the mean±s.e.m. of three independent experiments. ( c , d ) Neutrophils were stained at 3 dpf using the TSA kit, visualized by fluorescence microscopy and manually counted at the CHT. Each symbol represents one embryo and the mean±s.e.m. is also indicated. ( c ) stdMo, RNAas, n =17; TRMo2, RNAas, n =22; stdMo, RNAs, n =20; TRMo2, RNAs, n =19. ( d ) stdMo, RNAas, n =33; TRMo2, RNAas, n =30; stdMo, RNAs, n =35; TRMo2, RNAs, n =25. ( e ) Luciferase activity in tail sections of 2 dpf larvae. The graph shows the mean±s.e.m. of three independent experiments performed with triplicates samples. Statistical significance was assessed using the Student’s t -test ( P <0.05). Full size image We next decided to use a luciferase reporter assay in whole zebrafish embryos, as we have previously described [34] . The results showed that TR deficiency inhibited, while TR overexpression activated, gcsf promoter activity ( Fig. 6e ). Collectively, these results strongly suggest that TR regulate the expression of gcsf and mcsf genes which maintain a critical balance between the major myeloid ( spi1 ) and erythroid ( gata1 ) transcription factors. DC is an inherited disorder with mutations affecting telomerase components or telomere-stabilizing components, which is characterized by a variety of phenotypes [7] . However, DC patients usually die of bone marrow failure due to a deficient renewing capability of HSCs [8] , [9] . Curiously, the presentation of the disease is more serious in patients with mutations affecting TR [7] and some mutations, such as 58G→A, are not associated with impaired telomerase activity in vitro [35] . In addition, various lines of evidence have shown the cancer-promoting activity of TR independently of telomerase activity [17] , [18] , [19] , [20] . All these observations, together with the ability of TR to specifically bind 2,198 sites in the human genome [21] , led us to hypothesized that TR plays a non-canonical role in haematopoiesis through the regulation of gene expression. We found that genetic depletion of TR in zebrafish embryos with three different MOs resulted in a strong neutropenia and monocytopenia, which was fully rescued by the overexpression of TR RNA, confirming the specificity of the observed phenotype. Strikingly, the effect of TR in developmental myelopoiesis is independent of telomerase activity and telomere length, since tert mutant larvae showed normal number of neutrophils; TR depletion also led to neutropenia in tert mutant larvae; telomere length was weakly affected and to similar levels in TR - and tert -deficient larvae; and TR was expressed at very high levels in zebrafish neutrophils, while tert was undetectable in these cells. These results point to a non-canonical role of TR in myelopoiesis and suggest its probable involvement in the regulation of neutrophil function. This apparent discrepancy with TR -deficient mice, which do not show impaired myelopoiesis independently of telomere shortening, may be due to developmental and/or physiological compensations, which probably do not exist in humans [36] , [37] , [38] . TR -deficient neutrophils were recruited to wounds similarly to wild types. TR -deficient larvae did not show higher susceptibility to S. typhimurium and were able to upregulate il1b and tnfa genes at similar levels as wild types upon the infection. To the best of our knowledge, there is a single study on neutrophil function from DC patients [39] . This study showed that there was no significant difference in the degree of phorbol 12-myristate acetate (PMA) and N-formyl-methyonyl-leucyl-phenylalanine (fMLP)-triggered respiratory burst activity between 18 DC patients and their respective healthy family members. Unfortunately, the gene mutated in these patients was unknown and it is likely that there was a pool of patients with mutations affecting genes encoding different telomerase and/or telomere components. Our studies suggest that more DC patients should be examined for neutrophil defects. One of the most interesting observations of our study is that definitive haematopoiesis was not affected in TR -deficient embryos. Thus, the expression of canonical markers for EMPs and HSCs seemed to be normal, as the number of cd41 + cells at the CHT. Erythropoiesis and lymphopoiesis proceeded normally, further confirming that emergence, maintenance and differentiation of HSCs was unaffected in TR -deficient embryos. In contrast, TR -deficient embryos/larvae showed lower number of spi1 + and gcsfr + cells, confirming that TR is specifically required for the differentiation of myeloid cells, that is, neutrophils and macrophages. These results may explain the persistant neutropenia and altered myelopoiesis observed in DC children who showed normal erythropoiesis, megakaryopoiesis and normal lymphocyte subgroups and antibody levels [40] , [41] . We speculate that the critical role played by TR in telomere maintenance might have masked its non-canonical role in myelopoiesis, since the majority of DC patients are examined at later stages of the disease when critically short telomeres severely impair HSC renewal and bone marrow failure is imminent. Our in vivo genetic analysis provides the first experimental evidence to our knowledge that TR modulates a critical gene regulatory network required for myelopoiesis, probably by regulating the expression of the two main growth factors involved in the differentiation of neutrophils (Gcsf) and macrophages (Mcsf). This is not unexpected since human TR binds direct to both the CSF1 and CSF2 gene promoters [21] and there is a complex crosstalk between mouse GCSF/GMCSF and SPI1 (refs 42 , 43 , 44 ). Therefore, TR could act as a positive transcription factor for these genes. Although the direct binding of TR to gcsf and mcsf upstream regulatory sequences requires to be demonstrated, the subtle regulation of the zebrafish gcsf gene promoter by TR levels, assayed by a luciferase reporter assay in whole zebrafish larvae, supports this conclusion. The regulation of spi1 and gata1 genes in zebrafish has been shown to be critical for the differentiation of myeloid and erythroid cells. Reciprocal regulation of spi1 and gata1 determines myeloid versus erythroid fate [27] . In addition, loss of Gata1 transforms primitive blood precursors into myeloid cells, resulting in a massive expansion of granulocytic neutrophils and macrophages at the expense of red blood cells [45] . Our results demonstrate that TR modulates the myeloid versus erythroid fate outcomes from HSCs by differentially controlling the levels of spi1 and gata1 via upregulation of gcsf and mcsf . Intriguingly, transcription intermediate factor-1γ ( tif1g , trim33 ) also plays a similar role by differentially controlling the levels of spi1 and gata1 (ref. 46 ). The regulation of CSF genes by TR might have important clinical implications, since GCSF and GMCSF therapy has been used in DC patients to treat neutropenia [47] . It is tempting to speculate, therefore, that this therapy might be specifically efficient in DC patients carrying mutations in the TR gene before telomeres are critically short in HSC. While GCSF/GMCSF treatment has been found to be relatively effective in children [40] , [41] , [48] and young adults with DC [49] , [50] , in other cases the treatment was only moderately effective in improving neutropoiesis [51] , [52] . Unfortunately, the mutation responsible for DC in all these clinical trials was unknown. The different efficiency of GSCF/GMCSF therapy may be related to the mutated gene and the telomere length of the patients. This speculation is supported by the ability of CD34 + cells from DC patients with a TR mutation to produce the different lineages of mature cells in normal numbers in vitro in response to growth factors, despite the HSC compartment of these patients being profoundly reduced [53] . Taken together, these results further indicate that telomere dysfunction of HSCs from DC patients or knockout mice might unmask the non-canonical role of TR . In conclusion, this study provides experimental evidence that TR plays a non-canonical role in the regulation of myelopoiesis by fine-tuning the expression of spi1 and gata1 transcription factors in developing zebrafish embryos through the regulation of gcsf and mcsf . The in vivo model developed here is a powerful tool to illuminate the non-canonical functions of TR in HSC emergence, maintenance and differentiation. In this way, further studies with this model could elaborate signalling pathways that are perturbed in DC patients and could represent therapeutic targets. Ethics statement The experiments performed comply with the Guidelines of the European Union Council (86/609/EU). Experiments and procedures were performed as approved by the Bioethical Committee of the University Hospital ‘Virgen de la Arrixaca’ (Spain) and by the Children’s Hospital Boston institutional Animal Care and Use Committee (USA). Animals Zebrafish ( Danio rerio H., Cypriniformes, Cyprinidae) were obtained from the Zebrafish International Resource Center and mated, staged, raised and processed as described [54] . The tert mutant line (allele hu3430) was obtained from the Sanger Institute and has been previously described [28] , [55] . The casper mutant [56] and Tg( gata1 ::DsRed) [57] lines were previously described. The transgenics lines Tg( lyz ::DsRed) [25] , Tg( mpx ::eGFP) [24] , Tg( mpeg1 ::GAL4/ uas ::NTRmCherry) ( mpeg1 ::mCherry was used throughout this manuscript for clarity) [26] and Tg( cd41 ::eGFP) [31] were kindly provided by Drs P. Crosier, S. Renshaw, G. Lieschke and R.I. Handin, respectively. Morpholino and RNA injection Specific morpholinos (Gene Tools) were resuspended in nuclease-free water to 1 mM ( Supplementary Table 1 ). In vitro -transcribed RNA was obtained following the manufacturer’s instructions (mMESSAGE mMACHINE kit, Ambion). Both morpholinos and mRNA were mixed in microinjection buffer (0.5 × Tango buffer and 0.05% phenol red solution) and microinjected into the yolk sac of one- to eight-cell-stage embryos using a microinjector Narishige IM300 (0.5–1 nl per embryo). The amount of injected RNA is indicated in each figure. The same amount of MOs and RNA were used in all experimental groups. Analysis of development The effect of MOs on development was evaluated as previously reported [58] . Briefly, the side-to-side flexures were recorded at 22 hpf (25–26 somites stage). The heartbeat, red blood cells on yolk and early pigmentation in retina and skin were recorded at 24 hpf (Prim 5 stage). The head trunk angle (HTA), retina pigmentation, weak circulation, early touch reflect and, straight tail and caudal artery halfway to end of tail were recorded at 30 hpf (Prim 15 stage). The early motility, tail pigmentation, strong circulation, and caudal artery 3/4 of the way to the end of tail were recorded at 36 hpf (Prim 30 stage). Neutrophil staining Zebrafish embryos of different ages were fixed overnight at 4 °C in 4% paraformaldehyde (PFA) and neutrophils were specifically stained by using the TSA-Plus Fluorescein kit (Perkin Elmer), following the manufacturer’s instructions. Fluorescein-labelled neutrophils were then counted under an epifluorescence Lumar V12 stereomicroscope equipped with a digital camera (AxioCam MRm; Zeiss). Embryo blood collection and staining Blood cells were collected by cardiac puncture on anesthetized embryos in a solution of 0.02% tricaine (Sigma), 1% BSA in PBS, pH 7.4. Collected cells were immediately spread on glass slides, allowed to air dry, fixed in methanol for 30 s and stained by the Wright–Giemsa method [16] . o-dianisidine staining Embryos were anesthetized with tricaine at 2 dpf and stained with 1 mg ml −1 o-dianisidine (Sigma) in staining buffer (40% ethanol, 10 mM NaAc, 0.675% H 2 O 2 ) for 15 min in the dark. Flow cytometry Approximately 100–200 embryos were dechorionated with pronase (Roche), mechanically dissociated between 30 and 36 hpf through 100 and 70 μm cell strainers in 0.9 × PBS solution supplemented with 10% fetal calf serum (FCS). Cell suspensions were analysed by fluorescence-activated cell sorting (FACS) using a BD FACSCanto flow cytometer. Data analyses were performed using BD FACSDiva 6.1.3 software (BD Biosciences). Two- and 3-day tg( mpx :eGFP) larvae (300–600) were anesthetized in tricaine, minced with a razor blade, incubated at 28 °C for 30 min with 0.077 mg ml −1 Liberase (Roche) and the resulting cell suspension passed through a 40-μm cell strainer. eGFP + cells were then sorted using a staff-operated Beckman Coulter MoFlo Legacy Cell Sorter at the Bauer Core of the University of Harvard. Telomerase activity assay A real-time quantitative TRAP (Q-TRAP) analysis was performed [22] , [59] . Briefly, proteins were extracted from whole embryos/larvae using ice-cold NP-40 lysis buffer and real-time Q-TRAP performed with 0.1 and 1 μg protein extracts. For making the standard curve, a 1:10 dilution series of telomerase-positive sample (HeLa cells) was used. Control samples were obtained by treating the cell extracts with 1 μg RNase at 37 °C for 20 min. Data were collected and converted into Relative Telomerase Activity units performing the calculation: RTA of sample=10 (Ct sample − γint)/slope . The standard curve obtained was: y =−3.2295 x +23.802. Q-FISH Blood cells from 3 dpf larvae collected as described above were spread and hybridized with the PNA telomeric oligonucleotide (CCCTTA) 3 labelled with Cy3 (PE Biosystems) [60] . Cy3 and DAPI images were captured with × 100 and × 60 objectives respectively using a Nikon Digital Camera DXM 1200C on a Nikon Direct Eclipse fluorescence microscope. Telomere fluorescence signals were quantified using the TFL-TELO program (from Peter Lansdorp, Vancouver, Canada). Recruitment assay At 3 dpf, mpx ::GFP larvae were anesthetized in tricaine and complete transection of the tail was performed with a disposable sterile scalpel. Then, they were mounted in 1% (wt/vol) low-melting-point agarose dissolved in egg water. The success of transection was confirmed immediately through an epifluorescence Lumar V12 stereomicroscope equipped with green fluorescent filters. Each fish image was captured and established as zero time. Thereafter, images were captured at the selected times while animals were kept in their agar matrixes with the added medium at 28.5 °C. All images were acquired with the integrated camera on the stereomicroscope and were used for subsequently counting the number of neutrophils recruited to the wound area, established between the arterio-venous loop and the end of the tail. Bacterial infection assay Larvae were infected with ~10 CFU per larva of wild-type strain 12023 of Salmonella enterica serovar Typhimurium ( S. typhimurium ) kindly provided by Professor D.W. Holden. Briefly, bacteria were injected in the Duct of Cuvier of 2 dpf larvae and then monitored every 24 h over a 5-day period for clinical signs of disease and mortality [61] . Whole-mount RNA in situ hybridization Transparent Casper embryos were used for whole-mount RNA in situ hybridization [62] . lmo2 , spi1 ( pu.1 ), gata1a , gcsfr , cmyb , runx1 , rag1 , tert and tr RNA probes were generated using the DIG RNA Labelling Kit (Roche Applied Science) from linearized plasmids. Embryos were imaged using a Scope.A1 stereomicroscope equipped with a digital camera (AxioCam ICc 3, Zeiss). Analysis of gene expression Total RNA was extracted from whole embryos/larvae or sorted cell suspensions with TRIzol reagent (Invitrogen) following the manufacturer’s instructions and treated with DNase I, amplification grade (1 U μg −1 RNA; Invitrogen). SuperScript III RNase H − Reverse Transcriptase (Invitrogen) was used to synthesize first-strand cDNA with oligo(dT)18 (for all genes but TR ) or R1 (for TR ) primers from 1 μg of total RNA at 50 °C for 50 min. Real-time PCR was performed with a MyiQ instrument (BIO-RAD) using SYBR Premix Ex Taq (Perfect Real Time; Takara). Reaction mixtures were incubated for 10 min at 95 °C, followed by 40 cycles of 15 s at 95 °C, 1 min at 60 °C, and finally 15 s at 95 °C, 1 min at 60 °C, and 15 s at 95 °C. For each zebrafish mRNA, gene expression was normalized to the ribosomal protein S11 content in each sample using the comparative Ct method (2 − ΔΔ Ct ). The primers used are shown in Supplementary Table 3 . In all cases, each PCR was performed with triplicate samples and repeated at least with two independent samples. Analysis of gcsf gene promoter activity A 2 Kb genomic DNA sequence upstream of gcsf +1 position was amplified using the following primers: forward 5′-CAGTGTTGTGGTTTTGGTCCAGGCG-3′ and reverse 5′-CCGGACACCGAGCACCGGCGAGCCGCC-3′. The DNA fragment was cloned in the SmaI site of the pGL3basic vector (Promega) driving the expression of firefly luciferase gene ( gcsf ::Luc). One- to eight-cell-stage embryos were microinjected in the yolk with 0.5–1 nl of a mix containing 20 ng μl −1 of the firefly luciferase construct, 2 ng μl −1 of Renilla luciferase control plasmid, 1 ng per egg of stdMo and TRMo2 or 200 pg per egg of in vitro -transcribed TR RNA. After 48 h, tail sections of at least 50 larvae were obtained, pooled and assayed for luciferase activity using a Luminometer Optocomp I (MGM Instruments) [34] . Statistical analysis Data were analysed by analysis of variance (ANOVA). The differences between two samples were analysed by the Student’s t- test. A log rank test was used to calculate the statistical differences in the survival of the different experimental groups. How to cite this article: Alcaraz-Pérez, F. et al. A non-canonical function of telomerase RNA in the regulation of developmental myelopoiesis in zebrafish. Nat. Commun. 5:3228 doi: 10.1038/ncomms4228 (2014).